Prevalent and distinct spliceosomal 3′-end processing mechanisms for fungal telomerase RNA Telomerase RNA (TER) is an essential component of the telomerase ribonucleoprotein complex. The mechanism for TER 3′-end processing is highly divergent among different organisms. Here we report a unique spliceosome-mediated TER 3′-end cleavage mechanism in Neurospora crassa that is distinct from that found specifically in the fission yeast Schizosaccharomyces pombe . While the S. pombe TER intron contains the canonical 5′-splice site GUAUGU, the N. crassa TER intron contains a non-canonical 5′-splice site A UAAGU that alone prevents the second step of splicing and promotes spliceosomal cleavage. The unique N. crassa TER 5′-splice site sequence is evolutionarily conserved in TERs from Pezizomycotina and early branching Taphrinomycotina species. This suggests that the widespread and basal N. crassa -type spliceosomal cleavage mechanism is more ancestral than the S. pombe -type. The discovery of a prevalent, yet distinct, spliceosomal cleavage mechanism throughout diverse fungal clades furthers our understanding of TER evolution and non-coding RNA processing. The telomerase enzyme is responsible for the addition of telomeric DNA repeats onto the ends of eukaryotic chromosomes to maintain genome stability and cellular replicative capacity [1] . The core telomerase ribonucleoprotein (RNP) enzyme is composed of the catalytic telomerase reverse transcriptase (TERT) and telomerase RNA (TER) that contains a short region as the template for telomeric DNA repeat synthesis [2] . TERs are highly divergent across eukaryotic clades, differing immensely in nucleotide sequence, length and biogenesis pathway [3] , [4] . The diversity in TER biogenesis is evidenced by the different RNA polymerase (pol) machineries employed for transcription. While TER is transcribed by RNA pol II in most species, it is transcribed by RNA pol III in ciliates [5] , [6] , [7] , [8] . Furthermore, TERs from evolutionary separate groups of species associate with entirely unique groups of accessory proteins—the dyskerin complex and TCAB1 in vertebrates [9] , [10] ; Est1, Est3 and Sm-ring in budding yeasts [11] , [12] , [13] ; the dyskerin complex and POT1 in the plant Arabidopsis [14] , [15] and p50 and p65 in ciliates [16] . These separate sets of TER accessory proteins are essential for localization, RNP assembly and TER 3′-end processing [17] . The identification of the Schizosaccharomycetes pombe TER ( Spo TER1) revealed a spliceosome-mediated cleavage mechanism for RNA 3′-end processing [18] , [19] , [20] . The nascent Spo TER1 transcript harbours a downstream intron followed by a second exon and a 3′-poly(A) tail. The mature Spo TER1 3′-end is generated by spliceosomal cleavage at the 5′-splice site (5′-SS), removing the intron, second exon and poly(A) tail. This is in contrast to splicing—whereby the intervening intron sequence is excised and the neighbouring exons are joined [21] . The Spo TER1 intron itself uncouples these two tightly associated splicing steps by inhibiting the second transesterification step at the 3′-splice site (3′-SS). The second transesterification step is abated by a strong branch point sequence (BPS), an extended distance from the BPS to the 3′-SS and a weak polypyrimidine (Py) in the Spo TER1 intron [19] . Here we report in N. crassa a spliceosome-mediated mechanism for TER 3′-end processing that is distinct from the S. prombe -type. The N. crassa –type TER spliceosome-mediated 3′-end cleavage relies exclusively on a unique 5′-SS A UAAGU, which alone is necessary and sufficient for inhibiting the second transesterification step in splicing. This is the first biologically functional instance of spliceosome-mediated cleavage relying exclusively on the 5′-SS. In addition, the N. crassa -type TER intron is pervasive across Ascomycota , found universally in TERs from filamentous fungi and select early branching fission yeasts. This preponderance and conservation among distinct, evolutionary distant and basal fungal species suggest that this mechanism is more ancestral than the S. pombe -type. The discovery of a unique spliceosome-mediated cleavage mechanism provides new insights into TER biogenesis and evolution. Neurospora crassa TER precursor harbours an intron Neurospora crassa TER ( Ncr TER) was recently identified as a 2,049-nt RNA [22] . The 3′-end of the mature Ncr TER was determined by rapid amplification of cDNA ends (RACE) from total RNA treated with poly(A) polymerase ( Fig. 1a , lane 1). However, 3′-RACE with total RNA untreated with poly(A) polymerase generated two larger products ( Fig. 1a , lane 2). While the smaller of these two products was not readily visible by ethidium bromide staining, it was discernable for gel extraction. Cloning and subsequent sequencing of the two PCR products revealed distinct Ncr TER variants of ~400 and 470 nt in length. The 470-nt product harboured a 74-nt intron sequence, while the 400-nt product lacked this intron with the two exons joined ( Fig. 1b ). This intervening sequence contained the conserved features of a canonical intron: 5′-SS, BPS and 3′-SS ( Fig. 1c ). The presence of an intron in Ncr TER transcripts suggested that Ncr TER undergoes spliceosome-mediated cleavage for 3′-end processing, similar to that discovered in the fission yeast Spo TER1 (ref. 18 ). Interestingly, the Ncr TER intron 5′-SS A UAAGU is non-canonical, a stark contrast to the canonical 5′-SS GUAUGU sequence found in the Spo TER1 and mRNA introns [18] . We then determined the relative abundance of the three Ncr TER variants by performing northern blot analysis of total RNA with probes targeting either the first or second exon. The 2,049-nt Ncr TER was readily detected by northern blot, while the precursor and spliced variants were below the threshold for detection ( Fig. 1d ). This result suggests that the mature 2,049-nt Ncr TER variant has far greater abundance, which is consistent with our initial identification of only the 2,049-nt Ncr TER species in the purified telomerase holoenzyme [22] . 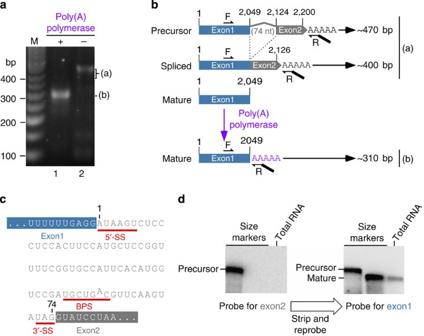Figure 1: Characterization of theNcrTER intron and 3′-end processing variants. (a) 3′-RACE ofNcrTER. Two distinct PCR products (a and b) were amplified from the RNA samples with (+) or without (−) poly(A) polymerase treatment. A 50-bp ladder (M) was included with sizes denoted. (b) Schematic ofNcrTER splicing variants. Exon 1 (blue box), 74-nt intron (grey line) and exon 2 (grey box) are denoted. Positions of forward (F) and reverse (R) primers used in RT-PCR are indicated. RT-PCR of the precursor and spliced RNA generated products (a) of 470 and 400 bp, respectively. RT-PCR of the matured RNA pretreated with poly(A) polymerase generated the 310 bp product (b). (c) Sequence of theNcrTER intron. The sequences of exon 1 (blue box) and exon 2 (grey box) flanking theNcrTER intron. The 5′-splice site (5′-SS), branch point sequence (BPS) and 3′-SS are denoted below the intron sequence. (d) Northern blot analysis ofNcrTER splicing variants. Northern blot was probed forNcrTER exon 2 (grey) first and the stripped blot was re-probed for exon 1 (blue).In vitrotranscribed precursor and matureNcrTER were loaded as size markers. Figure 1: Characterization of the Ncr TER intron and 3′-end processing variants. ( a ) 3′-RACE of Ncr TER. Two distinct PCR products (a and b) were amplified from the RNA samples with (+) or without (−) poly(A) polymerase treatment. A 50-bp ladder (M) was included with sizes denoted. ( b ) Schematic of Ncr TER splicing variants. Exon 1 (blue box), 74-nt intron (grey line) and exon 2 (grey box) are denoted. Positions of forward (F) and reverse (R) primers used in RT-PCR are indicated. RT-PCR of the precursor and spliced RNA generated products (a) of 470 and 400 bp, respectively. RT-PCR of the matured RNA pretreated with poly(A) polymerase generated the 310 bp product (b). ( c ) Sequence of the Ncr TER intron. The sequences of exon 1 (blue box) and exon 2 (grey box) flanking the Ncr TER intron. The 5′-splice site (5′-SS), branch point sequence (BPS) and 3′-SS are denoted below the intron sequence. ( d ) Northern blot analysis of Ncr TER splicing variants. Northern blot was probed for Ncr TER exon 2 (grey) first and the stripped blot was re-probed for exon 1 (blue). In vitro transcribed precursor and mature Ncr TER were loaded as size markers. Full size image Ncr TER-type intron is prevalent in Ascomycota fungal TERs Analysis of 72 additional Pezizomycotina filamentous fungal TERs that we previously identified revealed the absolute conservation of the Ncr TER-type intron in all species examined ( Fig. 2a ). All known Pezizomycotina TER introns contain the unique non-canonical 5′-SS A UAAGU sequence, the BPS sequence RCUR A Y that includes an invariant adenine residue as a putative branch point residue and the putative 3′-SS YAG ( Supplementary Fig. 1 ). The 3′-SS was experimentally verified by 3′-RACE for N. crassa , Aspergillus nidulans and Mycosphaerella graminicola ( Supplementary Fig. 1 ). The Ncr TER 5′-SS A UAAGU is extremely conserved in filamentous fungal TERs and distinct from the canonical, yet less conserved 5′-SS GURNGU found in yeast TER introns from the fission yeast S. pombe as well as species from the budding yeast Candida and Hansenula genera [18] , [23] , [24] . 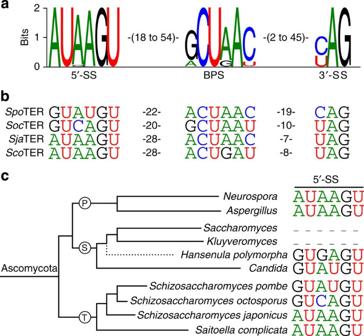Figure 2: Conservation and diversity of fungal TER intron sequence. (a) Sequence conservation of filamentous fungal TER introns. Consensus sequences of 5′-SS, BPS and 3′-SS are derived from a multiple sequence alignment of 73PezizomycotinaTER introns and presented using Sequence Logo. (b) Sequence conservation of fourTaphrinomycotinaTER introns. The aligned sequences of 5′-SS, BPS and 3′SS of TER introns fromSchizosaccharomyces pombe(Spo), S. octosporus(Soc),S. japonicus(Sja)andSaitoella complicata(Sco) are shown. (c) Evolutionary relationship of fungal TER introns. The phylogenetic tree of select species fromPezizomycotina(P),Saccharomycotina(S) andTaphrinomycotina(T) is based on a recent fungal six-gene phylogeny study (Jameset al. (2006); Liuet al. (2009)). Respective intron 5′-SS sequences from select species with known TER introns are shown. The length of the branch line does not reflect evolutionary distance. The evolutionary position ofHansenula polymorphais tentative (dashed line). Figure 2: Conservation and diversity of fungal TER intron sequence. ( a ) Sequence conservation of filamentous fungal TER introns. Consensus sequences of 5′-SS, BPS and 3′-SS are derived from a multiple sequence alignment of 73 Pezizomycotina TER introns and presented using Sequence Logo. ( b ) Sequence conservation of four Taphrinomycotina TER introns. The aligned sequences of 5′-SS, BPS and 3′SS of TER introns from Schizosaccharomyces pombe ( Spo), S. octosporus ( Soc) , S. japonicus ( Sja) and Saitoella complicata ( Sco ) are shown. ( c ) Evolutionary relationship of fungal TER introns. The phylogenetic tree of select species from Pezizomycotina (P), Saccharomycotina (S) and Taphrinomycotina (T) is based on a recent fungal six-gene phylogeny study (James et al . (2006); Liu et al . (2009)). Respective intron 5′-SS sequences from select species with known TER introns are shown. The length of the branch line does not reflect evolutionary distance. The evolutionary position of Hansenula polymorpha is tentative (dashed line). Full size image We then investigated whether the S. pombe-type or the N. crassa-type TER intron is more ancestral. S. pombe belongs to the subphylum Taphrinomycotina that together with the other two subphyla Pezizomycotina and Saccharomycotina constitute the Ascomycota phylum. In addition to TER that we previously cloned from the basal Taphrinomycotina species Saitoella complicata [22] , we identified two additional Taphrinomycotina TERs from Schizosaccharomyces octosporus and Schizosaccharomyces japonicus by a bioinformatics approach (see Methods). The 3′-ends and intron sequences of these newly identified TERs were experimentally determined by RACE. Surprisingly, there was a clear divide in the intron 5′-SS sequence among Taphrinomycotina TERs. The basal species S. complicate and S. japonicus harboured the N. crassa -type 5′-SS A UAAGU, while the later evolving species S. octosporus contained the S. pombe -type 5′-SS GURNGU ( Fig. 2b ). Thus, the more prevalent N. crassa -type intron appears to be more basal and thus ancestral than the S. pombe -type intron ( Fig. 2c ). Ncr TER-type 5′-SS promotes spliceosomal cleavage The 5′-SS of the Ncr TER and canonical mRNA introns differ with respect to their first and forth residues ( Fig. 3a ). Newman et al . [25] demonstrated in yeast that an introduced G-to-A substitution at the first residue in an mRNA intron suppresses the second step, yet permits the first step of splicing. We thus hypothesized that the 5′-SS is sufficient for Ncr TER 3′-end processing. To test this, we constructed a minimal exogenous expression cassette of the NcrTER gene. This minimal Ncr TER expression cassette spanned a 3′-portion (residues 1,888–2,049) of exon 1, the intron (residues 2,050–2,123), exon 2 (residues 2,124–2,200) and the 500 bp downstream flanking genomic sequence that contained a polyadenylation signal ( Fig. 3b,c ). This expression cassette also contained an eGFP gene as an internal control for RNA expression and normalization. Ncr TER and eGFP mRNA were transcribed independently under separate ccg-1 (clock-controlled gene-1) promoters and were fused to the ccg-1 5′-UTR sequence, generating ccg-1:: Ncr TER and ccg-1::eGFP, respectively. The ccg-1 promoter is a light induced, strong RNA pol II promoter commonly used for ectopic gene expression in the N. crassa model system [26] . Northern blot analysis was performed to determine the steady-state level of the Ncr TER exon 1 fragment and eGFP mRNA with probes targeting the fused ccg-1 5′-UTR sequence ( Fig. 3b ). The ccg-1:: Ncr TER construct generated a stable RNA product detectable by northern blot analysis ( Fig. 3d , lane 3). This RNA product had the expected 3′-end corresponding to the mature Ncr TER 3′-end, verified by 3′-RACE. Thus, the exogenous overexpressed minimal Ncr TER 3′-fragment was processed by spliceosome-mediated cleavage, similar to the full-length endogenous Ncr TER. RT-PCR was performed to detect the precursor and spliced RNA transcripts, which were below the detection limit of northern blot ( Figs 1d and 3d ). While the unspliced precursor and spliced Ncr TER 3′-fragments were both detected, the precursor appeared to be much more abundant ( Fig. 3e , lane 3). This is consistent with the RT-PCR results of the endogenous Ncr TER precursor and spliced product ( Fig. 1a , lane 2). Thus, our ccg-1:: Ncr TER expression cassette provides a minimal system for the functional analysis of spliceosome-mediated Ncr TER 3′-end processing. 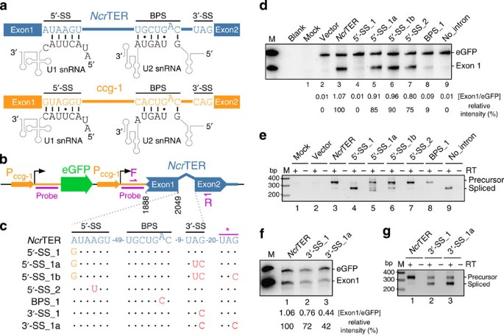Figure 3: Determinants in theNcrTER intron for spliceosomal cleavage. (a) Schematic of U1 and U2 snRNAs base-paired withNcrTER (top, blue) or ccg-1 (bottom, orange) intron 1. (b) Schematic of the dual gene cassette for expressing theNcrTER 3′-end fragment of exon 1, intron, exon 2 and 500 bp downstream sequence (blue) along with internal control eGFP (green) fused to the 5′-UTR of ccg-1 under theccg-1promoter (Pccg-1, orange) with the transcription initiation sites shown (black arrows). Annealing positions for riboprobes (Probe) as well as forward (F) and reverse (R) primers for RT-PCR are denoted (purple). (c) Alignment ofNcrTER intron mutations (red), mutations to convert theNcrTER intron into the ccg-1 mRNA intron (orange) and a downstream cryptic 3′-SS (*, purple) denoted. The accumulation and splicing variants produced from these intron mutations were evaluated by northern blot analysis (d,f) and RT-PCR (e,g). Relative intensity of spliceosomal cleaved ccg-1::NcrTER (Exon 1), determined by the ratio of Exon 1 over eGFP (Exon1/eGFP) with the background of each lane subtracted and relative to the wild-typeNcrTER intron, is shown below the blot and the markers (M) werein vitrotranscribed ccg-1::NcrTER Exon 1 and ccg-1::eGFP RNA. Figure 3: Determinants in the Ncr TER intron for spliceosomal cleavage. ( a ) Schematic of U1 and U2 snRNAs base-paired with Ncr TER (top, blue) or ccg-1 (bottom, orange) intron 1. ( b ) Schematic of the dual gene cassette for expressing the Ncr TER 3′-end fragment of exon 1, intron, exon 2 and 500 bp downstream sequence (blue) along with internal control eGFP (green) fused to the 5′-UTR of ccg-1 under the ccg-1 promoter ( P ccg-1 , orange) with the transcription initiation sites shown (black arrows). Annealing positions for riboprobes (Probe) as well as forward (F) and reverse (R) primers for RT-PCR are denoted (purple). ( c ) Alignment of Ncr TER intron mutations (red), mutations to convert the Ncr TER intron into the ccg-1 mRNA intron (orange) and a downstream cryptic 3′-SS (*, purple) denoted. The accumulation and splicing variants produced from these intron mutations were evaluated by northern blot analysis ( d , f ) and RT-PCR ( e , g ). Relative intensity of spliceosomal cleaved ccg-1:: Ncr TER (Exon 1), determined by the ratio of Exon 1 over eGFP (Exon1/eGFP) with the background of each lane subtracted and relative to the wild-type Ncr TER intron, is shown below the blot and the markers (M) were in vitro transcribed ccg-1:: Ncr TER Exon 1 and ccg-1::eGFP RNA. Full size image Mutations were introduced to the Ncr TER intron in 5′-SS, BPS and 3′-SS to identify the element(s) necessary for Ncr TER 3′-end processing ( Fig. 3c ). The 5′-SS_1 mutant with the first residue mutated from A to G reduced the level of mature Ncr TER exon-1 RNA to 8% of wild type ( Fig. 3d , lane 4), presumably by restoring the second step of splicing. Indeed, RT-PCR and subsequent sequencing of PCR products confirmed efficient splicing of the 5′-SS_1 mutant RNA ( Fig. 3e , lane 4; Supplementary Fig. 2 ). In contrast, the 5′-SS_2 mutant with the fourth residue mutated from A to U only slightly reduced the level of mature Ncr TER exon-1 RNA ( Fig. 3d , lane 7) and did not significantly affect splicing efficiency ( Fig. 3e , lane 7; Supplementary Fig. 2 ). Thus, the first adenosine residue in the Ncr TER 5′-SS appears to be the key determinant for Ncr TER 3′-end processing. We then examined if the 5′-SS_1 mutant—which has complete splicing restored—could be converted for S. pombe -type spliceosomal cleavage by extending the distance between the BPS and the 3′-SS ( Supplementary Fig. 3 ). We generated a double mutant 5′-SS_1a that, in addition to the 5′-SS_1 mutation, disrupted the 3′-SS ( Fig. 3c ). A triple mutant 5′-SS_1b further disrupted a downstream cryptic 3′-SS ( Fig. 3c ). Both 5′-SS_1a and 5′-SS_1b mutants effectively restored spliceosomal cleavage and accumulated mature RNA at levels comparable to the wild-type Ncr TER intron ( Fig. 3d , lanes 5 and 6), while reducing the splicing efficiency ( Fig. 3e , lanes 5 and 6). RT-PCR and sequencing of the spliced RNA products from 5′-SS_1a and 5′-SS_1b mutants showed that, when the preferred 3′-SS was mutated, two different cryptic 3′-SSs were used instead with low efficiencies ( Supplementary Fig. 2 ). Thus, disruption of the N. crassa -type spliceosomal cleavage in the 5′-SS_1 mutant was rescued by extending the distance between the BPS and the 3′-SS to employ S. pombe -type spliceosomal cleavage. To verify that the Ncr TER 3′-end processing is indeed spliceosome-mediated and not through non-specific endo- or exo-nucleolytic RNA degradation, we generated two mutations, BPS_1 and No_intron. Mutant BPS_1 abolished splicing by mutating the essential adenosine residue of the BPS and generated exclusively precursor RNA, while mutant No_intron produced only the corresponding spliced RNA product by deleting the entire intron. As expected, BPS_1 and No_intron mutants failed to accumulate mature RNA, indicating that spliceosome-mediated processing is required to generate the mature 3′-end of Ncr TER ( Fig. 3d , lanes 8 and 9). RT-PCR confirmed the lack of splicing with the BPS_1 mutant and the expected RNA transcript from the No_intron mutant ( Fig. 3e , lanes 8 and 9). The Ncr TER intron boundary 5′-AU/AG-3′ is chimeric with a 3′-SS similar to the canonical GU/AG mRNA introns and a 5′-SS similar to rare AU/AC mRNA introns [27] , [28] , [29] . We investigated whether the Ncr TER intron can be converted to an AU/AC intron for splicing. Mutations were introduced to convert the Ncr TER intron 3′-SS UAG to UAC. Mutant 3′-SS_1 had the proximal 3′-SS UAG changed to UAC, while mutant 3′-SS_1a had an additional mutation converting a downstream cryptic 3′-SS UAG to UAC ( Fig. 3c ). Mutant 3′-SS_1 showed a slightly decreased level of mature RNA at 80% of the wild type ( Fig. 3f , lane 2) and effectively increased splicing efficiency ( Fig. 3g , lane 2), confirmed by RT-PCR and sequencing of the spliced products ( Supplementary Fig. 2 ). Mutant 3′-SS_1a further decreased spliceosomal cleavage to 60% of the wild type ( Fig. 3f , lane 3) and a greater increase in splicing efficiency ( Fig. 3g , lane 3). Thus, the Ncr TER intron can be readily converted to an AU/AC splicing intron by mutating the proximal and distal 3′-SS UAG to UAC. 5′-SS AUAAGU converts an intron for spliceosomal cleavage The Ncr TER intron can be converted to favour splicing by a simple A-to-G substitution at the first adenine reside of the 5′-SS ( Fig. 3 ). To further confirm that the Ncr TER 5′-SS AUAAGU is the key determinate for spliceosomal cleavage, we performed a reciprocal experiment to convert an mRNA intron to the Ncr TER-type intron for spliceosomal cleavage. We modified our ccg1:: Ncr TER expression cassette by replacing the Ncr TER intron with an mRNA intron from the ccg-1 gene ( Fig. 4a ). 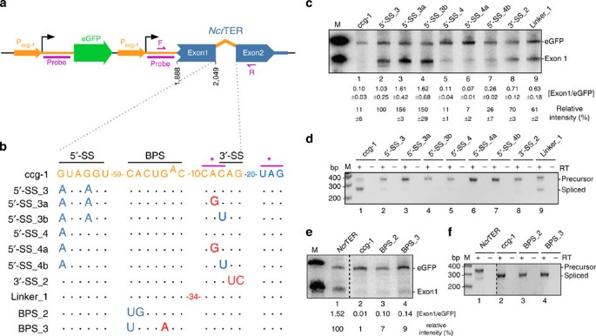Figure 4: Conversion of a ccg-1 mRNA intron to theNcrTER-type intron. (a) Schematic of the dual gene cassette for expressing the ccg-1::NcrTER (blue) with theNcrTER intron replaced with the ccg-1 mRNA intron (orange line). (b) Alignment of ccg-1 mRNA intron mutations (red), mutations to convert ccg-1 mRNA intron into theNcrTER-like intron (blue) and two cryptic 3′-SS (*, purple) denoted. The accumulation and splicing variants produced from these intron mutations were evaluated by northern blot analysis (c,e) and RT-PCR (d,f). Average relative intensity of two independent replicates with s.e. (c) and relative intensity (e) of spliceosomal cleaved ccg-1::NcrTER (Exon 1), determined by the ratio of Exon 1 over eGFP (Exon1/eGFP) with the background of each lane subtracted and relative to the mutant 5′-SS_3 or wild-typeNcrTER intron, is shown below the blot and the markers (M) werein vitrotranscribed ccg-1::NcrTER Exon 1 and ccg-1::eGFP RNA. Figure 4: Conversion of a ccg-1 mRNA intron to the Ncr TER-type intron. ( a ) Schematic of the dual gene cassette for expressing the ccg-1:: Ncr TER (blue) with the Ncr TER intron replaced with the ccg-1 mRNA intron (orange line). ( b ) Alignment of ccg-1 mRNA intron mutations (red), mutations to convert ccg-1 mRNA intron into the Ncr TER-like intron (blue) and two cryptic 3′-SS (*, purple) denoted. The accumulation and splicing variants produced from these intron mutations were evaluated by northern blot analysis ( c , e ) and RT-PCR ( d , f ). Average relative intensity of two independent replicates with s.e. ( c ) and relative intensity ( e ) of spliceosomal cleaved ccg-1:: Ncr TER (Exon 1), determined by the ratio of Exon 1 over eGFP (Exon1/eGFP) with the background of each lane subtracted and relative to the mutant 5′-SS_3 or wild-type Ncr TER intron, is shown below the blot and the markers (M) were in vitro transcribed ccg-1:: Ncr TER Exon 1 and ccg-1::eGFP RNA. Full size image Mutations were introduced to the ccg-1 mRNA at 5′-SS, BPS and 3′-SS to identify the element(s) necessary for conversion to Ncr TER-type spliceosomal cleavage ( Fig. 4b ). The replacement of the Ncr TER intron in our minimal expression cassette with the ccg-1 mRNA intron resulted in severely reduced spliceosomal cleavage ( Fig. 4c , lane 1) and markedly increased splicing efficiency ( Fig. 4d , lane 1). In mutant 5′-SS_3, replacing the ccg-1 5′-SS with the Ncr TER 5′-SS, by two G-to-A substitutions at the first and fourth positions of the 5′-SS, significantly increased the accumulation of mature Ncr TER exon-1 fragment ( Fig. 4c , lane 2) and reduced splicing efficiency ( Fig. 4d , lane 2). Thus, the Ncr TER 5′-SS AUAAGU alone appears to be sufficient to convert an mRNA intron for spliceosomal cleavage. Interestingly, sequencing the residual spliced products of the 5′-SS_3 mutant showed that a new 3′-SS CAC was utilized, similar to the AU/AC mRNA splicing introns ( Supplementary Fig. 4a ). In the presence of the 5′-SS AUAAGU, there is a shift from the 3′-SS YAG employed by GU/AG mRNA introns to YAC employed by AU/AC mRNA introns. To minimize the 3′-SS YAC, we generated two double mutants, 5′-SS_3a and _3b, that changed the 3′-SS CAC employed by mutant 5′-SS_3 to CGC or CAU, respectively ( Fig. 4b ). As expected, preventing AU/AC mRNA splicing for each of these mutants resulted in far greater accumulation of mature Ncr TER than the mutant 5′-SS_3 ( Fig. 4c , lanes 3 and 4) and similarly reduced splicing efficiency ( Fig. 4d , lanes 3 and 4). The residual spliced products from the mutants 5′-SS_3a and 5′-SS_3b arose from utilizing the 3′-SS CAG or UAG, respectively ( Supplementary Fig. 4a ). Thus, the 5′-SS_3a and 5′-SS_3b mutants employed the same 3′-SS YAG as the wild-type Ncr TER intron. We next investigated whether a single substitution at the first residue of the ccg-1 5′-SS would convert the ccg-1 mRNA intron to the Ncr TER intron. In contrast to mutant 5′-SS_3 that had both the first and fourth residues substituted and accumulated mature Ncr TER, mutant 5′-SS_4 with only the first residue substituted failed to accumulate mature Ncr TER above the level of the wild-type ccg-1 intron ( Fig. 4c , lane 5). The double mutations 5′-SS_4a and 5′-SS_4b eliminated the 3′-SS CAC to prevent AU/AC splicing. The northern blot showed that mutant 5′-SS_4a did not increase mature RNA level ( Fig. 4c , lane 6). However, mutant 5′-SS_4b had only a slight increase in mature Ncr TER accumulation, which is relatively insignificant compared with the 5′-SS_3 mutant ( Fig. 4c , lane 7). Thus, the ccg-1 mRNA intron requires a 5′-SS identical to the Ncr TER-type intron for spliceosomal cleavage. The requirement of G-to-A substitutions for the first and fourth residues in the ccg-1 mRNA intron may relay on the first adenine substitution disrupting snRNA U1 interaction and the fourth position substitution compensating for this disruption. As the ccg-1 mRNA intron can be easily converted into the Ncr TER-type intron, we examined whether the ccg-1 mRNA intron can be converted for the S. pombe -type spliceosomal cleavage by extending the distance between the BPS and 3′-SS CAG. Mutant 3′-SS_2 had the proximal 3′-SS eliminated, while mutant Linker_1 introduced a 34-nt insertion between the BPS and the 3′-SS CAG ( Fig. 4b ). The northern blot and RT-PCR results showed that both mutants had a significantly increased level of mature Ncr TER exon-1 RNA ( Fig. 4c , lanes 8 and 9) and decreased splicing efficiency ( Fig. 4d , lanes 8 and 9). Thus, the ccg-1 mRNA splicing intron can be readily converted to either the Ncr TER-type or Spo TER1-type intron for spliceosomal cleavage. We also examined the importance of the BPS in promoting spliceosomal cleavage. Mutant BPS_2 converted the ccg-1 mRNA intron BPS to Ncr TER-type intron BPS, while mutant BPS_3 converted it to the strong BPS of spo TER1 intron ( Supplementary Figs 3 and 4b ). These BPS mutants did not significantly increase the accumulation of mature Ncr TER ( Fig. 4e ) or decrease the splicing efficiency ( Fig. 4f ) compared with the wild-type ccg-1 mRNA intron. Telomerase biogenesis requires a 3′-end maturation step for TER, which is remarkably divergent across eukaryotic taxa and utilizes a wide array of distinct mechanisms. Within the phylum Ascomycota , certain budding yeast TERs employ specific transcription termination pathways and nucleolytic cleavage for 3′-end maturation [5] , [30] , while the fission yeast S. pombe and a few select budding yeast species employ spliceosomal cleavage [19] . Herein we have identified a second, yet vastly more widespread, spliceosome-mediated TER 3′-end processing mechanism initially in N. crassa and virtually ubiquitous throughout Ascomycete fungi. The N. crassa -type spliceosomal cleavage is mechanistically distinct from the S. pombe -type and is dependent on a unique 5′-SS A UAAGU sequence ( Fig. 2a and Supplementary Fig. 1 ). While critical for the S. pombe -type mechanism, the BPS and the distance to the 3′-SS are seemingly unimportant for the N. crassa -type. The prevalence of the N. crassa -type TER intron throughout all known Pezizomycotina fungal TERs and within the early diverging Taphrinomycotina fission yeast suggests that the N. crassa -type spliceosomal cleavage mechanism is ancestral and the S. pombe -type is later evolved. We propose that the highly prevalent and basal N. crassa -type TER intron is ancestral and the S. pombe -type intron is later evolved by an A-to-G substitution of the 5′-SS together with strengthening the BPS, extending distance to the 3′-SS and weakening the Py tract. It would seem less likely that multiple TER-intron fusion events occurred during the short evolutionary time within each of the three Ascomycete subphyla. Instead, it is more plausible that two transition events converted the N. crassa -type to the S. pombe -type intron independently along the fission and budding yeast lineages. The fission yeast transition event seems to have occurred adjacent to the emergence of the basal S. japonicas species that employs the ancestral N. crassa -type intron ( Fig. 5 ). Similarly, select budding yeast species from the genera Candida and Hansenula harbour the S. pombe -type intron for TER 3′-end maturation ( Figs 2c and 5 ), while later-branching budding yeast species appear to have lost the spliceosomal cleavage intron entirely. These Saccharomyces species with intron-less TERs instead employ the Nrd1/Nab3-dependent transcription termination pathway for generating non-polyadenylated TERs [30] . Two independent transition events from a more ancestral N. crassa -type TER intron to the S. pombe -type or the loss of TER intron explain the scattered presence of the S. pombe -type intron within Ascomycete fungal TERs and the uniform presence of the N. crassa -type intron. 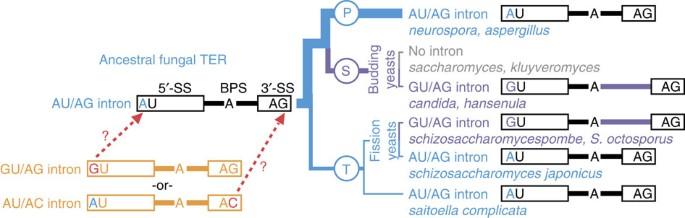Figure 5: An evolutionary history of the fungal TER intron. The AU/AG intron is predominate and basal (thick blue line) among fungal TER introns. The GU/AG or AU/AC (U1/U2-type) introns (orange) are the putative predecessor of the fungal TER AU/AG intron with only a single point mutation (red) in either intron necessary to convert into this intron type (dashed red lines). From this putative ancestral fungal TER AU/AG intron, the TER GU/AG type intron appears to have arisen twice independently (purple). A subgroup of budding yeasts has lost TER spliceosomal cleavage. Figure 5: An evolutionary history of the fungal TER intron. The AU/AG intron is predominate and basal (thick blue line) among fungal TER introns. The GU/AG or AU/AC (U1/U2-type) introns (orange) are the putative predecessor of the fungal TER AU/AG intron with only a single point mutation (red) in either intron necessary to convert into this intron type (dashed red lines). From this putative ancestral fungal TER AU/AG intron, the TER GU/AG type intron appears to have arisen twice independently (purple). A subgroup of budding yeasts has lost TER spliceosomal cleavage. Full size image While there is strong support for the ancestry of the N. crassa -type TER intron, there are two conceivable possibilities for the origin of the progenitor fungal TER intron. The progenitor fungal TER intron probably arose from a single gene fusion event between an intron-less fungal TER gene and either a common GU/AG or a rare AU/AC mRNA intron ( Fig. 5 ). This newly intron-containing TER gene then evolved into the N. crassa -type and later twice into the S. pombe -type TER intron. Deriving the N. crassa -type TER intron from a GU/AG intron requires alterations in the 5′-SS, while adoption from an AU/AC intron necessitates a C-to-G substitution of the last residue in the 3′-SS. Our mutagenesis studies demonstrate that the Ncr TER spliceosomal cleaving intron can be readily converted to either a canonical GU/AG or a rare AU/AC intron—permitting efficient splicing—with only single or double mutations necessary ( Figs 3 and 4 ). Previous studies in yeast have shown that an introduced G-to-A substitution of the first residue in the 5′-SS of a common GU/AG mRNA intron strongly inhibits the second step in splicing [25] , [31] . Arising from an AU/AC intron would negate a G-to-A transition substitution and instead require a 3′-SS mutation for efficient spliceosomal cleavage. Given the abundance of GU/AG mRNA intron in fungal genomes [32] , we favour the possibility that the N. crassa -type intron evolved from a GU/AG mRNA intron. While all three Ncr TER variants reconstituted equal telomerase activity in vitro ( Supplementary Fig. 5 ), it is evident that a spliceosomal cleaving TER intron is evolutionarily selected for as it removes the poly(A) tail from TER, which presumably prevents undesired cytoplasmic localization or poly(A) tail-mediated degradation [33] . Therefore, spliceosomal cleavage may promote nuclear retention and accumulation of functional TER. In S. pombe , disruption of TER spliceosome-mediated 3′-end processing results in reduced accumulation of Spo TER1 and telomere shortening [18] . The identification of additional fungal TERs from more basal species is necessary to determine the evolutionary origins of fungal TER introns. The identification of the widespread N. crassa -type spliceosomal cleavage mechanism within fungal TERs provides insights into the evolution of TER 3′-end processing. Spliceosomal cleavage was initially viewed as a molecular idiosyncrasy, unique to a single RNA from a single species. Our findings demonstrate that spliceosomal cleavage is the dominant mechanism for Ascomycete fungal TER 3′-end processing, found in the vast majority of species with known TERs. It has yet to be determined whether this mechanism is conserved outside of the Ascomycota phylum, due to the complete lack of TERs identified from the Basidiomycota phylum. Moreover, it is unlikely that this RNA processing mechanism is exclusive to TER and is potentially employed by other non-coding RNAs for 3′-end maturation. This work expands our understanding of the diversity of spliceosomal cleavage mechanisms, the origins and evolution of TER maturation, as well as our knowledge of non-coding RNA processing and biogenesis. Fungal strains N. crassa (FGSC 2489 wild type and FGSC 9720 NC1 his -3 mutant) and A. nidulans (FGSC A4 wild type) were obtained from the Fungal Genetics Stock Center (FGSC). N. crassa cells were grown at 30 °C with continuous light exposure in Vogel’s liquid minimal media supplemented with 2% sucrose [34] . A. nidulans cells were grown at 37 °C in YG liquid medium (0.5% yeast extract, 2% dextrose, 0.1% v/v Cove’s trace elements and 0.12% MgSO 4 ·7 H 2 O). M. graminicola cells (strain IPO323) were obtained from Dr Gert Kema and grown at 18°C in yeast glucose broth (1% yeast extract and 3% glucose). S. complicata (strain Y-17804), S. japonicus (strain Y-1361) and S. octosporus (strain Y-855) were obtained from ARS Culture Collection (NRRL) and grown at room temperature in YM broth (0.3% yeast extract, 0.3% malt extract, 0.5% peptone and 1% glucose). Identification of Schizosaccharomyces TER sequences Two protein-coding genes ( sub1 , SPAC16A10.03c and rho4 , dad1 ) flanking the SpoTER1 gene served as queries searching against S. japonicus (strain yFS275) and S. octosporus (strain yFS286) genomic sequencing data downloaded from the Broad Institute Database [35] . The intervening sequences between these putative protein coding genes were searched using the program Infernal [36] with a covariance model derived from the sequence alignment of Ascomycete TER three-way junctions [22] and yielded a unique hit for each species. The 5′- and 3′-ends of TERs from S. japonicus and S. octosporus were determined by RACE using the FirstChoice RLM-RACE kit (Life technologies). These cloned TER cDNAs sequences were deposited to GenBank with accession numbers KJ740640 ( S. japonicas ) and KJ740641 ( S. octosporus ). Generation of N. crassa recombinant strains The expression cassette containing the eGFP gene and the Ncr TER 3′-portion that includes exon-1 (residues 1,888–2,049), the 74-residue intron (residues 2,050–2,123), exon 2 (residues 2,124–2,200) and the 500 bp downstream flanking genomic sequence that contains a polyadenylation signal was constructed by overlapping PCR and cloned into the pCCG:: Ncr TER vector [22] , [37] . The eGFP gene and the Ncr TER 3′-portion were each fused immediately downstream of the ccg-1 5′-UTR and expressed under separate ccg-1 promoters. Intron mutants were generated by site-directed mutagenesis of this parental construct. For N. crassa transformation, the preserved conidia of N. crassa strain FGSC 9720 NC1 ( mat A his-3 Δmus-52::bar + ) were inoculated into 25 ml Vogel’s minimal solid media in a 500-ml flask. After growing at 30 °C for 3 days in total darkness, the mycelia were exposed to continuous light for 7 days. Conidia were harvested with 30 ml 1 M sorbitol and filtered through two layers of cheese cloth. Conidia were collected by centrifugation at 3,000 g for 3 min at 4 °C and washed three times with 1 M sorbitol. After the final wash the conidia were suspended in 1 M sorbitol to OD 600 of 0.5–1.0. Conidia were transformed with 1 μg of Stu I-linearized wild-type or mutant plasmid DNA by electroporation using a Gene Pulser Xcell system (Bio-Rad) set to 1,500 volts and 25 μF. Selection of his + transformants was performed in Vogel’s minimum medium supplemented with 2% sorbose in place of sucrose. Following growth at 30 °C for 3 days, the colonies were inoculated onto Vogel’s slants. Screening of homokaryon strains was performed by Southern blot analysis. Southern blot analysis Genomic DNA was isolated from 20 mg N. crassa mycelia using the Wizard Genomic DNA purification kit (Promega). The mycelia were lysed in 700 μl nuclei lysis solution in a 1.5 ml screw top tube containing 300 mg of 0.5-mm zirconia/silica beads (BioSpec Products) using a MiniBeadBeater-16 (BioSpec Products) at 3,450 r.p.m. for 1 min. The homogenates were incubated at 65 °C for 15 min and treated with 1 μl RNase A (50 mg ml −1 ) at 37 °C for 30 min. Following RNase treatment, 220 μl of protein precipitation buffer (Promega) was added, followed by vortexing vigorously for 20 s and incubation on ice for 5 min. After centrifugation at 16,000 g for 5 min, genomic DNA was precipitated by isopropanol and pelleted by centrifugation at 16,000 g for 1 min. The DNA pellet was washed once with 75% ethanol, air dried and suspended in 100 μl TE buffer (10 mM Tris-HCl pH 8.0 and 1 mM EDTA pH 8.0). Ten micrograms of genomic DNAs were digested with 10 U BspEI (New England Biolabs) in a 100 μl reaction at 37 °C overnight. Digested genomic DNA was phenol/chloroform extracted, ethanol precipitated and resolved on a 0.8% agarose gel. The agarose gel was denatured by immersion in a solution of 1.5 M NaCl and 0.5 M NaOH for 20 min twice, followed by neutralization in a solution of 1.5 M NaCl and 0.5 M Tris-HCl pH 7.5 for 15 min twice. The gel was dried in a gel dryer and pre-hybridized in 20 ml hybridization solution (5 × SSC, 5 × Denhardt’s reagent, 0.1% SDS and 20 mM NaH 2 PO 4 , pH 7.0) at 58 °C for 1 h. In-gel hybridization was performed at 58 °C overnight in 15 ml fresh hybridization solution with a 32 P end-labelled oligonucleotide probe targeting the his -3 locus. The gel was then washed at 58 °C for 20 min three times with a solution of 3 × SSC and 0.1% SDS and three times with a solution of 2 × SSC and 0.1% SDS. The gel was exposed to a phosphorstorage screen and imaged on a FX-Pro phosphorimager (Bio-Rad). Northern blot analysis Total RNA was isolated from N. crassa mycelia grown in Vogel’s minimum medium at 30 °C with continuous light exposure for expressing ccg1::eGFP and ccg1:: Ncr TER fusion genes under the light-inducible ccg-1 promoter. Twenty milligrams of mycelia were homogenized in 1 ml TRI-reagent (Molecular Research Center) at room temperature using 300 mg 0.5-mm zirconia/silica beads (BioSpec Products) and a MiniBeadBeater-16 (BioSpec Products) at 3,450 r.p.m. for 1 min. Homogenate was supplemented with 0.1 ml 1-bromo-3-chloropropane, vigorously mixed and centrifuged at 4 °C for phase separation. Residual phenol in the aqueous phase was removed by chloroform extraction followed by ethanol precipitation. For RNase H cleavage of ccg1::eGFP mRNA to remove the heterogeneous poly(A) tail, 16 μg total RNA was annealed with 600 pmol of DNA oligo (5′- AAGTCGTGCTGCTTCATGTG -3′) by incubation at 65 °C for 5 min and slowly cooled to room temperature. The RNA/DNA hybrid was digested with 5 U of RNase H (New England Biolabs) at 37 °C for 30 min followed by ethanol-precipitation. RNase H-treated total RNA was resolved on a 4% polyacrylamide/8 M urea gel, electrotransferred and UV crosslinked to a Hybond-XL membrane (GE Healthcare). For the full-length TER, untreated total RNA was resolved on a 1.5% agarose/formaldehyde denaturing gel, capillary transferred overnight and UV crosslinked to a Hybond-XL membrane (GE Healthcare). The membrane was pre-hybridized in ULTRAhyb hybridization buffer (Life technologies) at 65 °C for 30 min and hybridized overnight with a 32 P radio-labelled riboprobe targeting the ccg-1 5′-UTR fused to the eGFP mRNA and the Ncr TER 3′-fragment. The blot was washed at 65 °C twice in a solution of 1 × SSC and 0.2% SDS for 10 min, and twice in a solution of 0.2 × SSC and 0.1% SDS for 30 min. The blot was exposed to a phosphorstorage screen and imaged on a FX-Pro phosphorimager (Bio-Rad). RT-PCR Total RNA was treated with RNase-free DNase I (Zymo Research Corporation) to remove any genomic DNA contamination, followed by phenol/chloroform extraction and ethanol precipitation. For cDNA synthesis, 2 μg DNase I-treated total RNA was annealed with 100 pmol oligo d(T) 25 DNA primer in the presence of 10 pmol each dNTP by incubation at 65 °C for 3 min and quickly cooled on ice. A 20 μl reverse-transcription reaction was performed in 1 × Protoscript II Reverse Transcriptase Reaction buffer (50 mM Tris-HCl pH 8.3, 75 mM KCl and 3 mM MgCl 2 ), 10 mM DTT and 200 U ProtoScript II Reverse Transcriptase (New England Biolabs) at 48 °C for 30 min. The reaction was terminated by incubation at 80 °C for 5 min. PCR was performed in a 25-μl reaction with 1 μl of ½ × diluted reverse-transcription reaction in 1 × Q5 Reaction buffer (25 mM TAPS-HCl pH 9.3, 50 mM KCl, 2 mM MgCl 2 and 1 mM β-mercaptoethanol), 0.2 mM each dNTP, 0.5 U of Q5 DNA Polymerase, 0.2 μM forward primer (5′- CACAACACTCAAACCACTTTCAC -3′) and 0.2 μM reverse (5′- TGTTCGACACCGGTCACACT- 3′) primer. PCR products were resolved on a 3% agarose gel. The DNA bands corresponding to the spliced products were gel extracted using a Wizard SV gel and PCR clean-up system (Promega) and sequenced. How to cite this article: Qi, X. et al . Prevalent and distinct spliceosomal 3′-end processing mechanisms for fungal telomerase RNA. Nat. Commun. 6:6105 doi: 10.1038/ncomms7105 (2015). Accession codes: The sequences of S. japonicas and S. octosporus TERs were deposited to GenBank with accession numbers KJ740640 and KJ740641 , respectively.